Annexin A8 controls leukocyte recruitment to activated endothelial cells via cell surface delivery of CD63 To enable leukocyte adhesion to activated endothelium, the leukocyte receptor P-selectin is released from Weibel-Palade bodies (WPB) to the endothelial cell surface where it is stabilized by CD63. Here we report that loss of annexin A8 (anxA8) in human umbilical vein endothelial cells (HUVEC) strongly decreases cell surface presentation of CD63 and P-selectin, with a concomitant reduction in leukocyte rolling and adhesion. We confirm the compromised leukocyte adhesiveness in inflammatory-activated endothelial venules of anxA8-deficient mice. We find that WPB of anxA8-deficient HUVEC contain less CD63, and that this is caused by improper transport of CD63 from late multivesicular endosomes to WPB, with CD63 being retained in intraluminal vesicles. Consequently, reduced CD63 cell surface levels are seen following WPB exocytosis, resulting in enhanced P-selectin re-internalization. Our data support a model in which anxA8 affects leukocyte recruitment to activated endothelial cells by supplying WPB with sufficient amounts of the P-selectin regulator CD63. Vascular endothelial cells have a pivotal role in controlling blood vessel homeostasis. Upon activation through vessel damage or local inflammation, the endothelial surface is rapidly remodelled to an adhesive phenotype capable of capturing platelets and leukocytes. This remarkable change is brought about by the acute and rapid exposure of adhesive surface receptors, most importantly P-selectin and von Willebrand Factor (VWF), which recruit leukocytes and platelets. Together, these phenomena enable a strict temporal and spatial control of the adhesion cascade that leads to leukocyte extravasation into underlying inflamed tissue (for recent reviews see van Hinsbergh [1] and Pober and Sessa [2] ). P-selectin and VWF are stored in characteristic secretory organelles of endothelial cells, the Weibel-Palade bodies (WPB), that release their contents upon endothelial cell stimulation by secretagogues such as thrombin, histamine or vasopressin (for reviews, see Sadler [3] , Wagner [4] and Valentijin et al . [5] ). P-selectin externalization via regulated WPB exocytosis provides binding sites for P-selectin ligands on the leukocyte surface, initiating their tethering and rolling as a prerequisite for firm adhesion and subsequent extravasation. Recently, the tetraspanin CD63 (also known as lysosome-associated membrane protein 3 (LAMP3)) was shown to function as an essential cofactor for P-selectin-mediated leukocyte recruitment, presumably through stabilization of larger P-selectin clusters that are only formed in the presence of CD63 (ref. 6 ). In endothelial cells, the major pool of CD63 is found associated with late endosomes and lysosomes, where it is enriched on intraluminal vesicles (for review, see Pols and Klumperman [7] ). However, it is also present in WPB and at the cell surface [8] . Antibody uptake experiments revealed that plasma membrane CD63 is internalized to late endosomes and a fraction is then transported to WPB. Endothelial activation, in turn, leads to WPB exocytosis and cell surface presentation of CD63, indicating that this tetraspanin cycles between late endosomes and the plasma membrane via WPB [9] , [10] . Although lysosomal targeting signals were identified in the C-terminal cytoplasmic tail of CD63 and its endocytic transport to late endosomes/lysosomes is well characterized [11] , [12] , [13] , the trafficking route of endosomal CD63 to WPB is not clearly resolved, for example, with respect to the contribution of the trans-Golgi network or other intermediate compartments [10] , [14] . Considering the role of WPB-associated CD63 in P-selectin-mediated leukocyte adhesion, this transport process is, however, of prime importance, as it delivers CD63 to WPB and thus guarantees the simultaneous cell surface presentation of CD63 and P-selectin and their function in leukocyte recruitment [6] . Therefore, we set out to identify cellular factors required for the delivery of CD63 to WPB, focussing on endosome-associated components. Based on our previous finding showing that annexin A8 (anxA8) is required for late endosomal functions in non-polarized cells [15] , we hypothesized that this protein might participate in the delivery of CD63 from late endosomes to WPB. AnxA8 is a member of the annexin family of membrane-binding proteins that have been implicated in various membrane-trafficking steps. These include roles for anxA1 and anxA2 in the formation of late multivesicular endosomes (for reviews, see Futter and White [16] , and Gerke et al . [17] ) and for anxA8 in maintaining proper late endosome morphology and distribution, most likely by regulating the amount of endosome-associated actin [15] . Using human umbilical vein endothelial cells (HUVEC), we show here that anxA8 is required for the delivery of CD63 to WPB. As a consequence, ablation of anxA8 also reduces the levels of CD63 that are presented on the cell surface following endothelial stimulation while leaving the levels of acutely secreted VWF unchanged. This correlates with a reduction in P-selectin cell surface levels, an impaired leukocyte adhesion to anxA8-depleted endothelial cells and reduced leukocyte–endothelium interactions in inflammatory-activated anxA8-deficient mice. High-resolution imaging reveals that loss of anxA8 retains CD63 on the intraluminal vesicles of late multivesicular endosomes. Thus, anxA8 controls the pathway that ensures sorting and delivery of late endosomal CD63 to WPB and therefore efficient surface presentation of the P-selectin cofactor CD63 upon endothelial activation, which in turn is needed for leukocyte attraction. Endothelial anxA8 supports rolling and adhesion of human PMN Because anxA8 affects late endosome morphology and function in HeLa cells [15] and CD63 and P-selectin are thought to cycle through endosomes and then WPB to reach the endothelial cell surface following activation of WPB exocytosis [18] , we studied the effect of anxA8 on inflammatory P-selectin/CD63 functions. We ablated the protein in HUVEC using anxA8-specific small interfering RNA (siRNA) and non-targeting siRNA as control and examined the effect on primary human polymorphonuclear neutrophil (PMN) recruitment at physiological flow rates. Western blot analysis confirmed that levels of anxA8 were effectively and consistently reduced by 70–90%, whereas those of the unrelated gene product tubulin were unaffected ( Fig. 1a , Supplementary Fig. 7 ). When control siRNA-transfected HUVEC were exposed to histamine under flow conditions, adhesive interactions between PMN and HUVEC were readily observed, whereas these appeared strongly reduced in anxA8-depleted cells ( Fig. 1a , and also Supplementary Movies 1 and 2 ). To further substantiate these findings, the numbers of both rolling and adherent PMN as well as the rolling velocity of the cells were determined. HUVEC monolayers transfected with non-targeting control siRNA supported leukocyte interaction similar to that seen in non-transfected cells. In contrast, severely impaired PMN rolling and adhesion was seen on anxA8-depleted HUVEC ( Fig. 1b,c ). In all cases, PMN interactions with the activated HUVEC monolayer were dependent on the leukocyte receptor P-selectin, as they could be blocked with P-selectin-specific antibodies ( Fig. 1b,c ). Leukocytes did not roll and adhere via E-selectin, as the addition of anti-E-selectin antibodies able to block E-selectin-dependent leukocyte interaction with the endothelium ( Supplementary Fig. 1A ) had no effect ( Fig. 1b,c ), and no E-selectin could be detected on the surface of histamine-stimulated HUVEC ( Supplementary Fig. 1B , compare with lipopolysaccharide (LPS)-stimulated HUVEC). Leukocytes rolled on non-transfected and control siRNA-transfected HUVEC with comparable rolling velocities. In contrast, leukocyte rolling velocity was significantly increased on anxA8-depleted HUVEC ( Fig. 1d ). 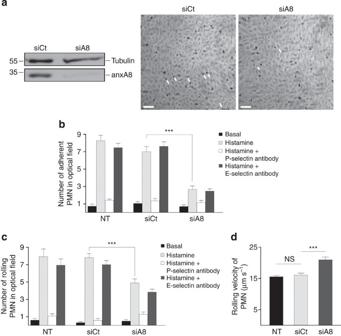Figure 1: Depletion of endothelial anxA8 impairs leukocyte rolling and adhesion. (a) Forty-eight hours after transfecting HUVEC with siRNA specific for anxA8 (siA8) or non-targeting siRNA (siCt), total cell lysates were prepared and analysed by immunoblotting using anti-anxA8 antibodies. α-Tubulin served as loading control (left panel). The right panel shows confluent HUVEC that were subjected to the same transfection regime and then placed in a parallel plate flow chamber and incubated with basal media or histamine-containing stimulation media for 20 min. The chambers were then perfused with isolated PMN for 7 min, while recording movies. The images shown represent the last section of the movies after histamine treatment of control and anxA8-depleted cells. Arrows mark firmly interacting leukocytes on the endothelial monolayers. Scale bars, 100 μm. Adhesion (b), rolling (c) and corresponding rolling velocities (d) of PMN on HUVEC monolayers of non-transfected (NT), siCt- or siA8-transfected cells were quantified and statistically analysed by one-way ANOVA followed by Tukey’s multiple comparison test. ***P<0.001. Data represent means±s.e.m. from at least 12 optical fields (b,c) or 31 rolling cells (d) from four independent experiments; AU, arbitrary units; NS, not significant. Figure 1: Depletion of endothelial anxA8 impairs leukocyte rolling and adhesion. ( a ) Forty-eight hours after transfecting HUVEC with siRNA specific for anxA8 (siA8) or non-targeting siRNA (siCt), total cell lysates were prepared and analysed by immunoblotting using anti-anxA8 antibodies. α-Tubulin served as loading control (left panel). The right panel shows confluent HUVEC that were subjected to the same transfection regime and then placed in a parallel plate flow chamber and incubated with basal media or histamine-containing stimulation media for 20 min. The chambers were then perfused with isolated PMN for 7 min, while recording movies. The images shown represent the last section of the movies after histamine treatment of control and anxA8-depleted cells. Arrows mark firmly interacting leukocytes on the endothelial monolayers. Scale bars, 100 μm. Adhesion ( b ), rolling ( c ) and corresponding rolling velocities ( d ) of PMN on HUVEC monolayers of non-transfected (NT), siCt- or siA8-transfected cells were quantified and statistically analysed by one-way ANOVA followed by Tukey’s multiple comparison test. *** P <0.001. Data represent means±s.e.m. from at least 12 optical fields ( b , c ) or 31 rolling cells ( d ) from four independent experiments; AU, arbitrary units; NS, not significant. Full size image The previous results suggested that anxA8-depleted HUVEC displayed a change in the P-selectin-mediated adhesive force, with the simplest explanation being reduced levels of P-selectin surface expression. To address this, we measured endothelial cell surface P-selectin using flow cytometry. 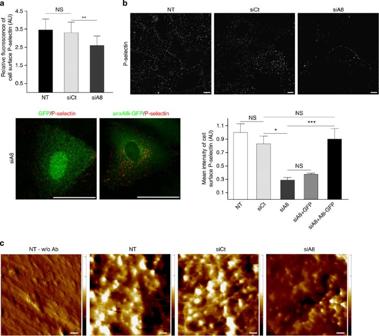Figure 2: Depletion of anxA8 reduces cell surface presentation of P-selectin. (a) HUVEC transfected as indicated were stimulated with histamine, incubated with fluorescently labelled anti-P-selectin antibodies and subsequently analysed by flow cytometry. MFIs of cell surface P-selectin of 10,000 cells were quantified. Statistical significance was evaluated by repeated measures ANOVA followed by Tukey’s multiple comparison test. **P<0.01; NS, not significant; bars represent means±s.e.m. from nine independent experiments. (b) Confocal imaging of histamine-induced cell surface P-selectin presentation of cells transfected as indicated (upper panel) or subjected to a second round of transfection using anxA8-specific siRNA together with a GFP expression vector (GFP) or a siRNA-insensitive anxA8 expression vector (anxA8i-GFP) 48 h after the initial transfection (lower panel). The cell surface pool of P-selectin was quantified by measuring MIFs in arbitrary units (AU). *P<0.05, ***P<0.001,P>0.05=NS; one-way ANOVA with Tukey’s multiple comparison test. Data represent means±s.e.m. from at least 15 single cells from four independent experiments. Scale bars, 10 μm. (c) HUVEC transfected as indicated were stimulated with histamine. Untreated cells (non-transfected (NT)—w/o Ab) and cells treated with anti-P-selectin antibodies were analysed by AFM to visualize the surface topology. Representative 10 × 10 μm deflection images of fixed cells obtained in contact mode in fluid are shown. Scale bars, 1 μm. Note that antibody-decorated HUVEC transiently transfected with anxA8 siRNA (siA8) show a smoother and less granular surface compared with non-transfected HUVEC (NT), as well as cells transfected with non-targeting siRNA (siCt). Figure 2a reveals that the amount of P-selectin on the cell surface of anxA8-depleted cells was significantly reduced as compared with control siRNA-transfected or non-treated cells. To confirm this, we directly visualized cell surface P-selectin by confocal microscopy and analysed the data by quantitative evaluation. As shown in Fig. 2b (upper panel), the punctate P-selectin staining pattern was significantly less prominent in anxA8-depleted HUVEC as compared with controls. We next verified that the reduced P-selectin cell surface presentation was attributed specifically to the loss of anxA8 by expressing green fluorescent protein (GFP) or a siRNA-insensitive anxA8i-GFP in anxA8-depleted HUVEC. As expected, in GFP-expressing cells the cell surface-associated P-selectin staining pattern remained low, whereas anxA8i-GFP completely restored the cell surface P-selectin levels ( Fig. 2b , lower panel). Figure 2: Depletion of anxA8 reduces cell surface presentation of P-selectin. ( a ) HUVEC transfected as indicated were stimulated with histamine, incubated with fluorescently labelled anti-P-selectin antibodies and subsequently analysed by flow cytometry. MFIs of cell surface P-selectin of 10,000 cells were quantified. Statistical significance was evaluated by repeated measures ANOVA followed by Tukey’s multiple comparison test. ** P <0.01; NS, not significant; bars represent means±s.e.m. from nine independent experiments. ( b ) Confocal imaging of histamine-induced cell surface P-selectin presentation of cells transfected as indicated (upper panel) or subjected to a second round of transfection using anxA8-specific siRNA together with a GFP expression vector (GFP) or a siRNA-insensitive anxA8 expression vector (anxA8i-GFP) 48 h after the initial transfection (lower panel). The cell surface pool of P-selectin was quantified by measuring MIFs in arbitrary units (AU). * P <0.05, *** P <0.001, P >0.05=NS; one-way ANOVA with Tukey’s multiple comparison test. Data represent means±s.e.m. from at least 15 single cells from four independent experiments. Scale bars, 10 μm. ( c ) HUVEC transfected as indicated were stimulated with histamine. Untreated cells (non-transfected (NT)—w/o Ab) and cells treated with anti-P-selectin antibodies were analysed by AFM to visualize the surface topology. Representative 10 × 10 μm deflection images of fixed cells obtained in contact mode in fluid are shown. Scale bars, 1 μm. Note that antibody-decorated HUVEC transiently transfected with anxA8 siRNA (siA8) show a smoother and less granular surface compared with non-transfected HUVEC (NT), as well as cells transfected with non-targeting siRNA (siCt). Full size image To visualize the cell surface distribution of P-selectin in stimulated and non-transfected, control siRNA- or anxA8 siRNA-transfected HUVEC at higher resolution, we used atomic force microscopy (AFM), as shown in Fig. 2c . Topographical inspection of the cell surface revealed that non-transfected cells displayed a rather smooth surface. Upon decoration with anti-P-selectin antibodies, the cell surface was now occupied by a fairly high number of globular structures that varied in size and most likely represented antibody-P-selectin complexes of different sizes. Antibody-decorated non-transfected and control siRNA-transfected cells shared a similar structural pattern. The surface of antibody-decorated, anxA8-depleted cells, however, was characterized by a lower density of globular structures. In addition, the globular structures on antibody-decorated cells depleted of anxA8 appeared smaller than those in non-transfected and control siRNA-treated cells, suggesting that clustering of cell surface P-selectin is reduced in the absence of anxA8. The rapid, stimulation-induced increase in P-selectin on the endothelial cell surface originates from WPB [19] , [20] . We therefore investigated whether the decrease in cell surface P-selectin observed in anxA8-depleted HUVEC was caused by less P-selectin being stored in WPB. Surprisingly, this was not the case; rather the P-selectin content was slightly but significantly increased ( Fig. 3a ). We next analysed whether the decrease in P-selectin cell surface presentation was caused by altered internalization rates and therefore visualized P-selectin internalization and intracellular trafficking by following the uptake of fluorescently labelled anti-P-selectin antibodies directed against the extracellular domain. Internalized P-selectin is transported to WPB [9] , [18] , and we observed that the amount of endocytosed anti-P-selectin antibodies that were delivered to WPB appeared to be slightly elevated in anxA8-depleted cells ( Fig. 3b ). These findings argue for a more rapid P-selectin internalization because of destabilized P-selectin clusters on the surface of cells lacking anxA8. To assess this more closely, we established an assay monitoring the uptake of anti-P-selectin antibodies by flow cytometry analysis. Cells were incubated with fluorescein-isothiocyanate (FITC)-labelled anti-P-selectin antibodies for 30 min at 37 °C to allow for antibody-bound P-selectin internalization and then treated with anti-FITC antibodies to quench the signal originating from non-internalized P-selectin remaining on the cell surface. Strikingly, anxA8-depleted cells accumulated more internalized signal as compared with controls ( Fig. 3c ). As these cells initially presented even less P-selectin on the surface ( Fig. 2 ), faster removal of P-selectin from their surfaces is likely to occur. 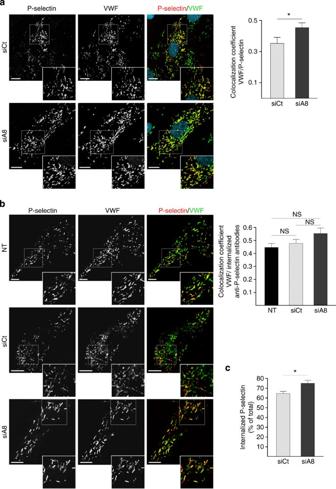Figure 3: AnxA8 depletion leads to increased internalization of P-selectin from the cell surface. (a) HUVEC transfected with control (upper panel) or anxA8-specific siRNA (lower panel) were co-stained with antibodies recognizing P-selectin (red) and VWF (green). Draq5 was used to label the nuclei. Colocalization coefficients (of VWF with P-selectin) from at least 23 images from five independent experiments were determined. Data are means±s.e.m. Scale bars, 10 μm. *P<0.05; unpaired Student’st-test. (b) Non-transfected HUVEC (NT) and HUVEC transfected with either non-targeting (siCt) or anxA8-specific siRNA (siA8) were cultivated for 48 h and then incubated in media containing antibodies against P-selectin for 24 h, fixed, permeabilized, incubated with the respective secondary antibodies and co-stained with antibodies against VWF. Scale bars, 10 μm. Colocalization coefficients of VWF with P-selectin antibodies from at least 13 individual cells from three independent experiments were determined as described in Methods. Statistical analysis was performed by one-way ANOVA followed by Tukey’s multiple comparison test.P>0.05=NS. (c) HUVEC transiently transfected with either non-targeting siRNA or anxA8-specific siRNA were allowed to internalize FITC-coupled anti-P-selectin antibodies at 37 °C for 30 min and subsequently analysed by flow cytometry. Relative fluorescence of internalized P-selectin was quantified and statistically analysed by unpaired Student’st-test. *P<0.05; data are means±s.e.m. from four independent experiments (10,000 cells per experiment). Figure 3: AnxA8 depletion leads to increased internalization of P-selectin from the cell surface. ( a ) HUVEC transfected with control (upper panel) or anxA8-specific siRNA (lower panel) were co-stained with antibodies recognizing P-selectin (red) and VWF (green). Draq5 was used to label the nuclei. Colocalization coefficients (of VWF with P-selectin) from at least 23 images from five independent experiments were determined. Data are means±s.e.m. Scale bars, 10 μm. * P <0.05; unpaired Student’s t -test. ( b ) Non-transfected HUVEC (NT) and HUVEC transfected with either non-targeting (siCt) or anxA8-specific siRNA (siA8) were cultivated for 48 h and then incubated in media containing antibodies against P-selectin for 24 h, fixed, permeabilized, incubated with the respective secondary antibodies and co-stained with antibodies against VWF. Scale bars, 10 μm. Colocalization coefficients of VWF with P-selectin antibodies from at least 13 individual cells from three independent experiments were determined as described in Methods. Statistical analysis was performed by one-way ANOVA followed by Tukey’s multiple comparison test. P >0.05=NS. ( c ) HUVEC transiently transfected with either non-targeting siRNA or anxA8-specific siRNA were allowed to internalize FITC-coupled anti-P-selectin antibodies at 37 °C for 30 min and subsequently analysed by flow cytometry. Relative fluorescence of internalized P-selectin was quantified and statistically analysed by unpaired Student’s t -test. * P <0.05; data are means±s.e.m. from four independent experiments (10,000 cells per experiment). Full size image Taken together, the impaired ability of anxA8-depleted HUVEC to interact with leukocytes is most likely because of a reduced surface presentation of P-selectin, which in turn is caused by a more rapid internalization. AnxA8 regulates CD63 levels on the cell surface and in WPB Recently, the secretagogue-induced cell surface presentation of P-selectin was reported to critically depend on the tetraspanin CD63 (ref. 6 ). Thus, the lower P-selectin cell surface presentation observed upon anxA8 depletion might be caused by reduced CD63 cell surface levels. To examine this possibility, we visualized CD63 on the surface of histamine-stimulated HUVEC by confocal immunomicroscopy. Strikingly, the cell surface signal of CD63 was drastically lower in anxA8-depleted cells than in controls ( Fig. 4a ). As CD63 is internalized from the cell surface, and a fraction of this internalized CD63 is transported from endosomes to WPB, thereby supplying the maturing WPB with CD63 (refs 10 , 14 , 18 ), we next measured the colocalization of the WPB marker protein VWF with CD63 in anxA8-depleted compared with control cells. As shown in Fig. 4b , quantitative analysis revealed that in contrast to the slightly increased presence of P-selectin in WPB ( Fig. 3 ), there was significantly less CD63 present in WPB of anxA8-depleted HUVEC. To confirm that the reduced CD63 amount in WPB was attributed specifically to the loss of anxA8, we performed rescue experiments. As expected, expression of anxA8i-GFP in anxA8-depleted HUVEC restored the colocalization of CD63 and VWF to control levels ( Supplementary Fig. 2 , and compare with Fig. 4b ). 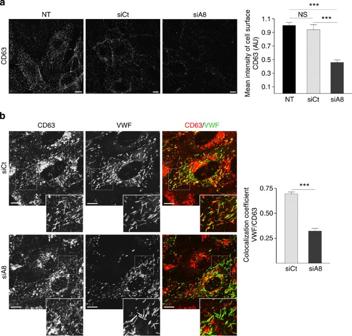Figure 4: AnxA8 depletion results in reduced levels of CD63 on the cell surface and in WPB. (a) Non-transfected HUVEC (NT) as well as HUVEC transiently transfected with either anxA8-specific siRNA (siA8) or non-targeting siRNA (siCt) were subjected to histamine-containing medium for 20 min, and then stained with anti-CD63 antibodies (left). The mean levels of anti-CD63 immunoreactivity presented on the cell surface were quantified by measuring fluorescence intensities in arbitrary units (AU; right). ***P<0.001,P>0.05=NS; one-way ANOVA with Tukey’s multiple comparison test; data represent means±s.e.m. of at least 17 images from four independent experiments. (b) HUVEC transfected with non-targeting siRNA (upper panel) or anxA8-depleted HUVEC (lower panel) were co-stained with antibodies against CD63 (red) and VWF as a marker for WPB (green). Colocalization coefficients (of VWF with CD63) from at least 47 individual cells from three independent experiments were then determined. Data are means±s.e.m. ***P<0.0001; unpaired Student’st-test. Scale bars represent 10 μm. Figure 4: AnxA8 depletion results in reduced levels of CD63 on the cell surface and in WPB. ( a ) Non-transfected HUVEC (NT) as well as HUVEC transiently transfected with either anxA8-specific siRNA (siA8) or non-targeting siRNA (siCt) were subjected to histamine-containing medium for 20 min, and then stained with anti-CD63 antibodies (left). The mean levels of anti-CD63 immunoreactivity presented on the cell surface were quantified by measuring fluorescence intensities in arbitrary units (AU; right). *** P <0.001, P >0.05=NS; one-way ANOVA with Tukey’s multiple comparison test; data represent means±s.e.m. of at least 17 images from four independent experiments. ( b ) HUVEC transfected with non-targeting siRNA (upper panel) or anxA8-depleted HUVEC (lower panel) were co-stained with antibodies against CD63 (red) and VWF as a marker for WPB (green). Colocalization coefficients (of VWF with CD63) from at least 47 individual cells from three independent experiments were then determined. Data are means±s.e.m. *** P <0.0001; unpaired Student’s t -test. Scale bars represent 10 μm. Full size image The results presented above suggested that the reduced CD63 cell surface presentation seen in anxA8-depleted cells was because of inefficient recruitment of CD63 to WPB. Thus, anxA8 most likely affects the transport of CD63 from endosomes to WPB and it could do so by acting either at the level of late endosomes as the donor organelle of CD63 or at the level of WPB as the acceptor granule. To determine the likely site of action, we expressed anxA8 fused to GFP and visualized its subcellular distribution in HUVEC. AnxA8-GFP did not show any overlap with WPB (visualized by VWF staining; Supplementary Fig. 3A ), but localized mainly to vesicular structures that stained positive for lysobisphosphatidic acid (LBPA) ( Supplementary Fig. 3B ), a poorly degradable phospholipid found in multivesicular late endosomes [21] , [22] . AnxA8-GFP also colocalized with the late endosomal pool of CD63 ( Supplementary Fig. 3C ). In accordance with our previous data obtained in HeLa cells [15] , the anxA8-GFP-positive late endosomes were sometimes enlarged. Overexpression or downregulation ( Supplementary Figs 3A and 4A ) of anxA8 did not affect the morphology or intracellular distribution of WPB. Ablating anxA8 also seemed to have no impact on the global maturation of WPB, as the small GTPase Rab27a that is recruited to only mature WPB [23] displayed normal WPB-localization in anxA8-deficient HUVEC ( Supplementary Fig. 4A ). Furthermore, subcellular fractionation by discontinuous sucrose gradient centrifugation revealed that WPB from anxA8-depleted HUVEC show the same fractionation characteristics and VWF content as WPB from control-transfected cells. Of interest, fractions containing the majority of VWF appeared slightly but consistently shifted in gradients from anxA8-depleted cells, suggestive of an altered protein to lipid ratio, and the major VWF peak had less CD63, again indicating that WPB in cells lacking anxA8 contain less CD63 ( Supplementary Fig. 4B,C ). In contrast to this effect on the CD63 loading of WPB, depletion of endothelial anxA8 did not affect the secretion competence of WPB, as release of VWF upon stimulation with histamine was the same in both anxA8-depleted and control cells ( Supplementary Fig. 4D ). Thus, while anxA8 affects the amount of WPB-associated CD63, it seems unlikely that it acts at the level of WPB; rather multivesicular late endosomes appear to be the site of anxA8 action. Trafficking of CD63 from endosomes to WPB depends on anxA8 To determine whether anxA8 is indeed involved in mediating the transfer of internalized CD63 to WPB, we next analysed CD63 dynamics in living HUVEC that expressed VWF fused to GFP as a marker protein for WPB. Internalization and intracellular trafficking of CD63 were visualized by following the uptake of fluorescently labelled antibodies directed against the CD63 extracellular domain for 4 h after antibody addition. This experimental setup was reported to selectively record CD63 cycling from the plasma membrane via late endosomes to WPB, as antibodies against late endosomal components not found in WPB were not transported to the WPB [10] . In control siRNA-transfected cells, we detected a clear colocalization of WPB and antibody signals for internalized CD63 as early as 3 h after the addition of antibodies ( Fig. 5a and Supplementary Movie 3 ). In contrast, anxA8-depleted cells did not show any distinct colocalization of internalized anti-CD63 antibodies with labelled WPB even 4 h after internalization, although the total amount of internalized antibodies appeared to be unaffected ( Fig. 5a and Supplementary Movie 4 ). It was previously shown that the highest amount of internalized anti-CD63 antibodies is found in WPB 24 h post antibody addition [10] . In accordance, at this time point we detected a considerable fraction of the internalized antibodies in the WPB of control cells, indicative of an efficient transfer of the internalized CD63 to WPB. However, the amount of internalized anti-CD63 antibodies detected in WPB after 24 h was considerably lower in anxA8-depleted cells, and quantitative analysis of the colocalization between internalized anti-CD63 antibodies and VWF revealed a significant reduction in anxA8-depleted cells as compared with controls ( Fig. 5b ). This effect was not observed in HUVEC, in which a related annexin, anxA2, had been depleted by siRNA ( Supplementary Fig. 5 ), arguing for a specific effect of anxA8 on the CD63 import into WPB. 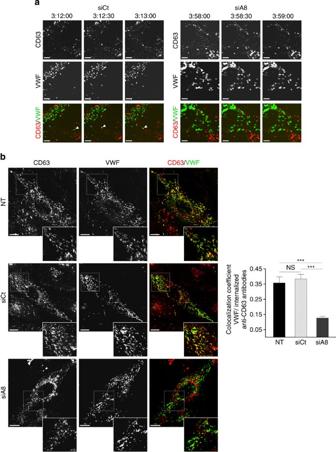Figure 5: Transport of internalized anti-CD63 antibodies to WPB is affected in anxA8-depleted HUVEC. (a) HUVEC cotransfected with VWF-GFP (green) and either non-targeting siRNA (siCt) or anxA8-specific siRNA (siA8) were incubated with anti-CD63 antibodies directly coupled to TRITC (red). One hour after antibody addition, cells were monitored in intervals of 30 s for 3 h. Three individual frames of each movie are shown. Arrowheads indicate colocalization of WPB and internalized CD63 antibodies. Scale bars, 5 μm. (b) HUVEC, non-transfected or transfected with either control or anxA8-specific siRNA, were incubated for 24 h in media containing antibodies against CD63, fixed, permeabilized, incubated with the respective secondary antibodies and co-stained with antibodies against VWF. Scale bars, 10 μm. Colocalization coefficients of VWF with CD63 from at least 16 individual cells from three independent experiments were determined as described in Methods. ***P<0.001,P>0.05=NS; one-way ANOVA with Tukey’s multiple comparison test. Data represent means±s.e.m. Figure 5: Transport of internalized anti-CD63 antibodies to WPB is affected in anxA8-depleted HUVEC. ( a ) HUVEC cotransfected with VWF-GFP (green) and either non-targeting siRNA (siCt) or anxA8-specific siRNA (siA8) were incubated with anti-CD63 antibodies directly coupled to TRITC (red). One hour after antibody addition, cells were monitored in intervals of 30 s for 3 h. Three individual frames of each movie are shown. Arrowheads indicate colocalization of WPB and internalized CD63 antibodies. Scale bars, 5 μm. ( b ) HUVEC, non-transfected or transfected with either control or anxA8-specific siRNA, were incubated for 24 h in media containing antibodies against CD63, fixed, permeabilized, incubated with the respective secondary antibodies and co-stained with antibodies against VWF. Scale bars, 10 μm. Colocalization coefficients of VWF with CD63 from at least 16 individual cells from three independent experiments were determined as described in Methods. *** P <0.001, P >0.05=NS; one-way ANOVA with Tukey’s multiple comparison test. Data represent means±s.e.m. Full size image As our findings strongly argued for a direct effect of anxA8 on CD63 trafficking, we used structured illumination microscopy (SIM) to more precisely resolve the subcellular localization of CD63 ( Fig. 6a ). Upon internalization, CD63 travels via early endosomes to the multivesicular late endosomal/lysosomal compartment, in which the majority of CD63 is sorted onto intraluminal vesicles [7] . As anxA8 is also found on multivesicular late endosomes of HUVEC ( Supplementary Fig. 3B ), we asked whether depletion of anxA8 might interfere with the sorting of CD63 within the multivesicular endosomes. Knocking down anxA8 did neither change the amount of the late endosomal/lysosomal protein LAMP2, which resides in the single limiting membrane of multivesicular late endosomes [7] ( Supplementary Fig. 6A ), nor that of CD63 ( Supplementary Fig. 6B ) in this compartment. This argues against a general disturbance of the membrane protein distribution in multivesicular late endosomes following anxA8 depletion. However, intraluminal CD63 signals appeared more intense in anxA8-depleted cells ( Fig. 6a ), and quantitative analysis revealed that anxA8-depleted HUVEC displayed a significantly higher ratio of intraluminal versus limiting membrane-associated CD63, the latter being identified by colocalization with LAMP2 ( Fig. 6b ). This argues for a sorting defect of CD63 within the multivesicular endosomes of the anxA8-depleted cells, which in turn disturbs proper transport of CD63 to WPB. 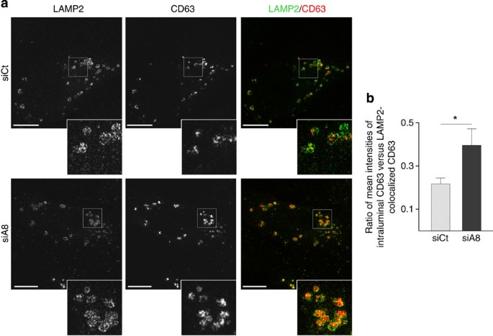Figure 6: Localization of CD63 to internal vesicles of late endosomes is increased in anxA8-depleted HUVEC. (a) HUVEC transiently transfected with non-targeting siRNA (siCt) or siRNA specific for anxA8 (siA8) were co-stained with antibodies against LAMP2 (green) and CD63 (red). Image stacks of single cells were recorded by super-resolution structured illumination microscopy. Scale bars, 10 μm. (b) LAMP2 signals over threshold were used as a mask to measure the CD63 signal intensity at the limiting membrane of endolysosomes. Ratios of mean intensities of CD63 on intraluminal membranes to CD63 at the limiting membranes were calculated as described in Methods for at least 12 images from three independent experiments. *P<0.05; unpaired Student’st-test. Figure 6: Localization of CD63 to internal vesicles of late endosomes is increased in anxA8-depleted HUVEC. ( a ) HUVEC transiently transfected with non-targeting siRNA (siCt) or siRNA specific for anxA8 (siA8) were co-stained with antibodies against LAMP2 (green) and CD63 (red). Image stacks of single cells were recorded by super-resolution structured illumination microscopy. Scale bars, 10 μm. ( b ) LAMP2 signals over threshold were used as a mask to measure the CD63 signal intensity at the limiting membrane of endolysosomes. Ratios of mean intensities of CD63 on intraluminal membranes to CD63 at the limiting membranes were calculated as described in Methods for at least 12 images from three independent experiments. * P <0.05; unpaired Student’s t -test. Full size image AnxA8 knockout mice show defects in leukocyte rolling and adhesion To verify the impact of anxA8 on leukocyte recruitment to inflammatory-activated endothelial cells in vivo , we generated anxA8 knockout mice (anxA8 KO) utilizing Cre-LoxP strategy. Therefore, we first established a homozygous mouse line in which exon 2 of the ANXA8 gene was flanked by LoxP sites. These mice (fl/fl) were then crossed with the pgk-Cre strain, which uniformly expresses the Cre site-specific recombinase, leading to Cre-mediated deletion of the floxed exon 2 in all tissues of offspring ( Fig. 7a–d ). Immunoblotting of tail tissue lysates from these KO (fl/fl;pgk-Cre) mice as compared with wild-type (wt; +/+) mice revealed the absence of anxA8 protein in the KO animals, whereas expression of the closely related anxA2 was unaffected ( Fig. 7e , Supplementary Fig. 7 ). We next analysed leukocyte rolling and adhesion in the inflamed cremaster muscle of the anxA8 KO mice and their heterozygous littermates (+/fl;pgk-Cre) as controls. Intravital microscopy revealed that both leukocyte rolling and adhesion to inflammatory-activated postcapillary venules were significantly impaired in KO mice as compared with control animals ( Fig. 8a–c , and Supplementary Movies 5 and 6 ). This phenotype was accompanied by a significant increase in leukocyte rolling velocity ( Fig. 8d ). AnxA8 is not expressed in murine leukocytes [24] , and we found that surface levels of the P-selectin counterligand P-selectin glycoprotein ligand-1 (PSGL-1), which is constitutively expressed on neutrophils, were unchanged in the anxA8 KO mice ( Fig. 8e ). This strongly suggests that the activated postcapillary venule endothelium of anxA8 KO mice exhibits an impaired ability to support leukocyte rolling and adhesion, resembling our observations in anxA8-depleted HUVEC. 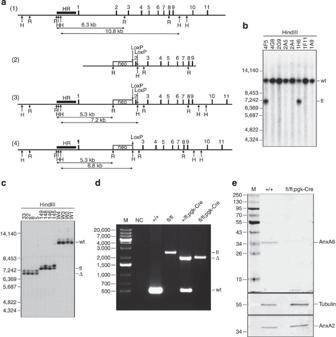Figure 7: Conditional deletion of theANXA8allele. (a) (1)ANXA8wt locus; (2) targeting vector (without negative selection marker and plasmid backbone); (3) genomic locus after homologous recombination (intron 1 containing the neomycin cassette, LoxP-flanked exon 2); (4) after removal of exon 2 by crossing with a pgk-Cre mouse. Numbered filled boxes represent exons, and lines represent intronic and intergenic regions. The empty box corresponds to the neomycin resistance cassette (neo) flanked by the FRT sites (not shown). Arrows indicate the LoxP sequences, and EcoRI (R) and HindIII (H) restriction sites. The black box represents the Southern probe (HR). (b) Southern blot analysis of ES cell colonies. Clones 1H6 and 4F5 contain the targeted (fl)ANXA8gene. (c) Southern blot analysis of tail biopsy DNA isolated from wt (W1, W2, W3 and W4),ANXA8targeted (fl; 145, 146, 148 and 149), andANXA8exon 2-deleted (Δ; 5, 8, 22 and 33) animals. Additional small bands are because of incomplete digestion at the left HindIII site and hence generation of fragments extended by 261 bp. (d) Genotyping PCR on tail genomic DNA. M, molecular weight standard; NC, negative control PCR without genomic DNA; +/+, wt animals; fl/fl, homozygous animals carrying theANXA8floxed allele; +/fl;pgk-Cre, offspring after crossing homozygous targeted animals with pgk-Cre mice; fl/fl;pgk-Cre, homozygous KO mice. (e) Detection of anxA8 protein expression in wt (+/+) and KO (fl/fl;pgk-Cre) mice by immunoblotting. α-Tubulin served as loading control. Note that expression of anxA2 is unchanged. Figure 7: Conditional deletion of the ANXA8 allele. ( a ) (1) ANXA8 wt locus; (2) targeting vector (without negative selection marker and plasmid backbone); (3) genomic locus after homologous recombination (intron 1 containing the neomycin cassette, LoxP-flanked exon 2); (4) after removal of exon 2 by crossing with a pgk-Cre mouse. Numbered filled boxes represent exons, and lines represent intronic and intergenic regions. The empty box corresponds to the neomycin resistance cassette (neo) flanked by the FRT sites (not shown). Arrows indicate the LoxP sequences, and EcoRI (R) and HindIII (H) restriction sites. The black box represents the Southern probe (HR). ( b ) Southern blot analysis of ES cell colonies. Clones 1H6 and 4F5 contain the targeted (fl) ANXA8 gene. ( c ) Southern blot analysis of tail biopsy DNA isolated from wt (W1, W2, W3 and W4), ANXA8 targeted (fl; 145, 146, 148 and 149), and ANXA8 exon 2-deleted (Δ; 5, 8, 22 and 33) animals. Additional small bands are because of incomplete digestion at the left HindIII site and hence generation of fragments extended by 261 bp. ( d ) Genotyping PCR on tail genomic DNA. M, molecular weight standard; NC, negative control PCR without genomic DNA; +/+, wt animals; fl/fl, homozygous animals carrying the ANXA8 floxed allele; +/fl;pgk-Cre, offspring after crossing homozygous targeted animals with pgk-Cre mice; fl/fl;pgk-Cre, homozygous KO mice. ( e ) Detection of anxA8 protein expression in wt (+/+) and KO (fl/fl;pgk-Cre) mice by immunoblotting. α-Tubulin served as loading control. Note that expression of anxA2 is unchanged. 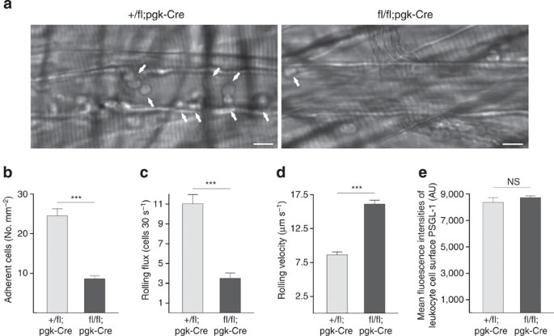Figure 8: Leukocyte rolling and adhesion is impaired in anxA8 KO mice. (a) Cremaster muscles were prepared from anxA8 KO mice (fl/fl;pgk-Cre) as well as from heterozygous littermates (+/fl;pgk-Cre). The number of adherent leukocytes (b), leukocyte rolling flux (c) and corresponding rolling velocity (d) were determined by transillumination intravital microscopy of blood vessels in the Cremaster. Scale bars, 10 μm. Leukocyte numbers were determined from at least 18 movies (four individuals per condition) of different postcapillary venules (b,c). (d) Rolling velocities of at least 60 rolling leukocytes were analysed in the respective intravital movies. Statistical analysis was performed by unpaired Student’st-test; ***P<0.001. (e) Murine whole-blood samples from anxA8 KO mice as well as from heterozygous littermates were analysed for PSGL-1 surface expression on leukocytes by flow cytometry. Bars represent means±s.e.m. from at least 900 leukocytes per mouse. Statistical analysis was performed by unpaired Student’st-test.P>0.05=NS. Full size image Figure 8: Leukocyte rolling and adhesion is impaired in anxA8 KO mice. ( a ) Cremaster muscles were prepared from anxA8 KO mice (fl/fl;pgk-Cre) as well as from heterozygous littermates (+/fl;pgk-Cre). The number of adherent leukocytes ( b ), leukocyte rolling flux ( c ) and corresponding rolling velocity ( d ) were determined by transillumination intravital microscopy of blood vessels in the Cremaster. Scale bars, 10 μm. Leukocyte numbers were determined from at least 18 movies (four individuals per condition) of different postcapillary venules ( b , c ). ( d ) Rolling velocities of at least 60 rolling leukocytes were analysed in the respective intravital movies. Statistical analysis was performed by unpaired Student’s t -test; *** P <0.001. ( e ) Murine whole-blood samples from anxA8 KO mice as well as from heterozygous littermates were analysed for PSGL-1 surface expression on leukocytes by flow cytometry. Bars represent means±s.e.m. from at least 900 leukocytes per mouse. Statistical analysis was performed by unpaired Student’s t -test. P >0.05=NS. Full size image In this study, we show that anxA8 controls P-selectin-dependent leukocyte recruitment to activated endothelial cells by supplying WPB with sufficient amounts of the P-selectin cofactor CD63. Within minutes after pro-inflammatory activation, P-selectin is expressed on the endothelial cell surface [19] , [20] . This acute surface presentation of P-selectin is not seen on endothelial cells of VWF KO mice that cannot form WPB and show both, strongly reduced cell surface expression of P-selectin and decreased leukocyte recruitment, even though the amount of intracellular P-selectin remains unchanged [25] . The defect in P-selectin cell surface presentation observed in these mice indicates that the rapidly releasable pool of P-selectin originates from WPB and emphasizes the importance of these specialized secretory organelles as P-selectin storage compartments in the control of inflammation [25] , [26] , [27] . We observed that anxA8-depleted HUVEC displayed a severe reduction in leukocyte rolling and adhesion upon histamine activation. This was accompanied by significantly reduced cell surface levels of P-selectin that could be restored upon re-expression of RNAi-resistant anxA8. Surprisingly, the WPB-associated P-selectin content in anxA8-depleted cells was slightly elevated. This can be explained by our findings of a more rapid P-selectin endocytosis and higher amounts of anti-P-selectin antibodies being delivered to WPB, indicating that in anxA8-depleted cells, P-selectin transport from the plasma membrane to WPB was enhanced. How could the changes in P-selectin cell surface presentation and re-internalization observed in the absence of anxA8 be brought about? Recent evidence indicates that CD63, another WPB component, acts as a P-selectin retention factor at the plasma membrane. Ablation of CD63 was reported to cause decreased P-selectin levels at the cell surface, resulting in impaired leukocyte recruitment [6] . Indeed, we found that levels of CD63 were significantly reduced on the plasma membrane of anxA8-silenced cells when the cells had been stimulated with histamine. Contrary to the increased presence of P-selectin in WPB, we found strongly decreased amounts of CD63 in WPB of anxA8-depleted HUVEC. These findings point to a regulatory function of anxA8 in delivering CD63 to WPB, which is in line with the suggestion that WPB-derived CD63 stabilizes cell surface levels of P-selectin [6] . The fact that we did not detect any effects of either increased or reduced levels of anxA8 on the formation, overall morphology or regulated exocytosis of WPB (defined by the histamine-evoked release of VWF) argues against a contribution of direct VWF–PMN interactions [28] to the impaired leukocyte recruitment seen in anxA8-ablated HUVEC. The trafficking pathways of CD63 in endothelial cells appear to be rather complex, with CD63 cycling between the plasma membrane and WPB via endosomal compartments [10] . Experimental evidence indicates that the CD63 present in WPB originates from late endosomes that are typically multivesicular and contain luminal vesicles surrounded by the limiting membrane [10] , [14] , [18] . CD63-specific antibodies are internalized and travel through the early and then the late endosomal compartments before eventually reaching the WPB [10] . Likewise, internalized anti-P-selectin antibodies can be found in WPB following transport through endosomes [9] . However, differences appear to exist between the transport of endosomal CD63 and P-selectin to WPB. P-selectin is delivered to newly forming WPB already at the level of the trans-Golgi network, whereas CD63 is only recruited to the secretagogue-responsive, mature WPB [10] , [14] . This is in line with our antibody uptake experiments in anxA8-depleted cells that revealed a defect in the transport of CD63, leading to diminished CD63 levels in WPB, while transfer of P-selectin to WPB remained unaltered. Although the existence of such transport routes from late endosomes to the secretory pathway seems quite evident, the mechanism and the late endosomal components responsible for delivery of CD63 to WPB are mostly uncharacterized, and the relation between late endosomes and WPB remains to be established. Within the multivesicular late endosomes, CD63 is found enriched on the intraluminal vesicle membrane as compared with the limiting membrane [7] . We hypothesized that anxA8 could affect the sorting of CD63 within the multivesicular endosomes, which in turn is required for proper transport of CD63 to WPB. Indeed, our results show that anxA8 depletion causes an increase of intraluminal CD63 at the expense of CD63 in the limiting membrane. As the latter is most likely the relevant pool for WPB transport, missorting in the absence of anxA8 will affect WPB transport of CD63. It remains to be determined how anxA8 that is associated with the cytosolic face of the limiting late endosomal membrane controls intraendosomal sorting of CD63. An obvious explanation would be a direct interaction that could increase the amount of CD63 in the limiting membrane. However, we were not able to obtain evidence for a direct interaction in co-immunoprecipitation experiments performed following cell lysis with different detergents. Although this negative result does not fully rule out the possibility of a direct interaction, we favour the notion of an indirect effect whereby anxA8 provides a late endosomal membrane scaffold that associates with membrane components embedding CD63. This would be in line with the molecular action of other annexins functioning as membrane scaffold at different target membranes [17] . Another member of the annexin family, anxA2, was also shown to affect WPB biology as its depletion strongly interfered with VWF release [29] , [30] . However, our results revealed that anxA2 ablation did not inhibit CD63 trafficking, suggesting that it might rather have a regulatory role in WPB exocytosis and not in endosome-to-WPB transport. Thus, different annexins may act sequentially on the multistep process leading to WPB maturation and the release of their stored components. To prevent autoimmunity/inflammatory disorders, immune homeostasis, that is, the rapid but reversible conversion between an anti-adhesive endothelium and an endothelium with enhanced leukocyte adhesiveness, must be ensured. Thus, the precise tempo-spatial regulation of endothelial surface adhesion molecules is of key importance, and it is conceivable that this is achieved through the superimposition of several layers of regulation. Our data support a model in which anxA8-dependent delivery of CD63 from multivesicular late endosomes to WPB critically controls P-selectin presentation on activated endothelial cells. This establishes the anxA8-controlled trafficking route of CD63 as vitally important for the regulation of major factors mediating efficient leukocyte/endothelium interactions as also revealed by the compromised leukocyte adhesiveness seen in the inflammatory-activated anxA8 KO mouse. Further analysis is required to reveal the molecular machinery operating on the still poorly characterized endosome-to-WPB transport pathway. Antibodies and plasmids Mouse monoclonal anti-human VWF antibodies (clone F8/86; 1:200), rabbit polyclonal anti-human VWF antibodies (1:200, 1:1,000 for enzyme-linked immunosorbent assay (ELISA)) and peroxidase-conjugated rabbit polyclonal anti-human VWF antibodies (1:8,000) were obtained from Dako (Glostrup, Denmark). Sheep anti-human VWF antibodies (1:200), FITC-coupled sheep anti-human VWF antibodies (1:500) and mouse monoclonal anti-FITC antibodies (1:20) were purchased from Abcam (ab112511, Cambridge, UK). Mouse monoclonal antibodies against human CD63 (1:600) and LAMP2 (1:50; clones H5C6, H4B4) were from the Developmental Studies Hybridoma Bank (University of Iowa, Iowa City, IA, USA), mouse monoclonal anti-Rab27a antibodies (sc-74586; 1:100) and mouse monoclonal antibodies against CD63 conjugated to tetramethylrhodamine isothiocyanate (TRITC) (sc-5275; 1:5) from Santa Cruz Biotechnology (Heidelberg, Germany), mouse monoclonal antibodies against α-tubulin (clone B-1-5-2; 1:5,000) from Sigma-Aldrich (St. Louis, MO, USA), and rabbit polyclonal antibodies against human anxA8 from Acris (AP00292PU-N, Herford, Germany; 1:500). Polyclonal rabbit antibodies raised against recombinant mouse anxA8 were a kind gift from Torsten Stein (Cancer Research UK Glasgow Centre, University of Glasgow). Mouse monoclonal anti-P-selectin antibodies (556087; 1:100) and rat monoclonal anti-PSGL-1 antibodies (clone 2PH1, PE-conjugated; 1:200) were obtained from BD Biosciences (San Diego, CA, USA) and mouse monoclonal antibodies against E-selectin were from R&D Systems (BBA26, Minneapolis, MN, USA; 25 μg ml −1 ). Sheep polyclonal antibodies against P-selectin (AF 137; 1:300, 1:100 for surface staining, 25 μg ml −1 for leukocyte adhesion assay), and sheep IgG isotype control (5-001-A) from R&D Systems were either used uncoupled or conjugated to FITC (Thermo Scientific; 8 ng μl −1 ) or DyLight 488 (Thermo Scientific; 2.5 ng μl −1 ). The mouse monoclonal anti-anxA2 antibody HH7 (1:1,000) has been described previously [31] . Mouse monoclonal antibodies used for the detection of LBPA (clone 6C4; 1:50) [21] were kindly provided by Jean Gruenberg (University of Geneva, Geneva, Switzerland) and mouse monoclonal antibodies used for the visualization of internalized CD63 (clone 1B5; 1:300; 1:100 for surface staining) [32] were a kind gift from Mark Marsh (University College London). Rat UZ4 monoclonal antibodies used for the detection of surface E-selectin (1:2) were kindly provided by Rupert Hallmann (University Hospital Münster, Germany) [33] . Secondary anti-mouse antibodies coupled to Alexa Fluor 488 (1:400) or Alexa Fluor 568 (1:400) were obtained from Molecular Probes (Eugene, OR, USA); horseradish peroxidase-conjugated anti-mouse or anti-goat antibodies (1:2,000) were obtained from Dako (Hamburg, Germany); TRITC-conjugated secondary anti-sheep antibodies (1:200) and anti-mouse antibodies coupled to Cy5 (1:100) were obtained from Jackson ImmunoResearch (Newmarket, Suffolk, UK). For the development of western blots using infrared detection, secondary IRDye 800 CW-conjugated goat anti-rabbit antibodies (1:10,000) and IRDye 680 CW-conjugated goat anti-mouse antibodies (1:10,000) were purchased from LI-COR (Bad Homburg, Germany). The mammalian expression construct for GFP-tagged anxA8 had been described previously [34] . For rescue experiments, a siRNA-insensitive mutant (anxA8i) was generated by introducing seven silent mutations into the siRNA-targeted region of the anxA8 cDNA. VWF-EGFP containing an internal GFP replacing the A2 domain of VWF [35] was a kind gift from Jan Voorberg (Sanquin Research, Amsterdam). Cell culture, transfection and RNAi HUVEC cultivated on CellBind Surface dishes (Corning) or on collagen type 1-coated coverslips were maintained in endothelial cell growth medium (PromoCell) at 37 °C in 7% CO 2 . HUVEC were transfected using the Amaxa Nucleofection Technology (HUVEC Nucleofector Kit-OLD, Lonza) according to the manufacturer’s instructions. Following transfection, cells were cultured for 48 h (siRNA) or for 24 h (plasmid). To trigger regulated secretion, cells were treated with 100 μM histamine (Sigma-Aldrich) for 20 min in basal medium (M-199; PAA, Pasching, Austria) containing 0.5% BSA, 100 U ml −1 penicillin and 100 μg ml −1 streptomycin. siRNA-mediated depletion of anxA8 was achieved by transfecting HUVEC with 200–400 pmol siRNA (5′-GGAGCGAGAUUGACUUAAAdTdT-3′) [15] . Control experiments used non-targeting siRNAs (AllStars negative control siRNA; Qiagen, Valencia, CA, USA). For rescue experiments, 48 h after the initial siRNA transfection, cells were transfected with anxA8-specific siRNA together with a siRNA-insensitive anxA8-GFP expression construct. Leukocyte adhesion assay PMNs were isolated from human whole blood using Histopaque gradients according to the manufacturer’s protocol (Sigma-Aldrich). HUVECs were transfected with anxA8-specific or control siRNAs, grown to confluency on a 35-mm tissue culture dish, and then stimulated with 20 μM histamine at 37 °C for 20 min or 1 nM interleukin-1β (IL-1β) for 4 h. PMN rolling and adhesion were determined using a parallel plate flow chamber assembly (Glycotech, Gaithersburg, MD, USA) perfused with isolated PMN (1 × 10 6 cells ml −1 ) at a constant shear stress of 0.7 dyne cm −2 for 7 min. Movies were obtained with an inverted TS100 transmission light microscope (Nikon) equipped with a × 10/0.25 objective and a digital camera (Pixelfly, Cooke Corporation, Romulus, MI, USA). Rolling and adherent cells were analysed using ImageJ software (NIH, Bethesda, MD, USA). Rolling velocity, given as μm s −1 , was calculated by measuring the time required for a cell to roll across the distance covered in the optical field. For antibody blocking experiments, anti-P-selectin (AF 137, R&D Systems) or anti-E-selectin antibodies (BBA26, R&D Systems) were incubated with the HUVEC for 30 min at 37 °C and added to the perfusion media at a concentration of 25 μg ml −1 . Immunofluorescence HUVEC destined for immunofluorescence labelling were fixed with 4% paraformaldehyde (PFA)/PBS for 10 min at room temperature and subsequently permeabilized using 0.2% Triton X-100/PBS for 2 min at room temperature. In the case of anxA8-GFP-expressing HUVEC, cells were fixed using cold methanol (−20 °C) for 3 min and then 4% PFA/PBS for 10 min at room temperature. After blocking with 2% BSA/PBS for 30 min at room temperature, samples were incubated with primary and the appropriate secondary antibodies, each applied for 1 h at room temperature. For surface staining of proteins (CD63, P-selectin), cells were first incubated with the appropriate primary antibodies for 2 h at 4 °C, fixed in 4% PFA/PBS for 15 min at 4 °C, permeabilized in 0.2% Triton X-100/PBS for 2 min at room temperature, and then incubated with the respective secondary antibodies for 1 h at room temperature. Confocal microscopy was carried out using a LSM 510 or LSM 710 META microscope (Carl Zeiss, Jena, Germany) both equipped with a Plan-Apochromat 63x/1.4 oil immersion objective. For the quantification of VWF/CD63 or VWF/P-selectin colocalization, digital images were imported into BioImageXD [36] , and fluorescent signals for VWF and CD63 or P-selectin were thresholded. Subsequently, colocalization coefficients were calculated using the BioImageXD colocalization tool. Analysis of CD63 and P-selectin surface localization used ImageJ software (NIH). Antibody internalization HUVEC were transfected with anxA8-specific (siA8) or control siRNAs (siCt) and then grown on collagen-coated coverslips for 48 h. Mouse monoclonal antibodies against CD63 (clone 1B5) were added, and cultivation was continued for another 24 h. Cells were then fixed with 4% PFA/PBS, permeabilized, and subjected to indirect immunofluorescence. For live cell approaches, HUVEC were transfected with the VWF-GFP plasmid and anxA8-specific or control siRNAs and then grown in collagen-coated labtecs for 48 h. Subsequently, specific anti-CD63 antibodies directly coupled to TRITC (sc-5275, Santa Cruz Biotechnology) were added. Labtecs were then placed on the microscope stage of a LSM 710 META microscope maintained at 37 °C and 7% CO 2 and imaged using a Plan-Apochromat × 63/1.4 oil immersion objective. Flow cytometry analysis of P-selectin and PSGL-1 For quantitative measurements of P-selectin cell surface pools, HUVEC were incubated with DyLight488-coupled anti-P-selectin antibodies at 4 °C for 30 min. To quantify P-selectin internalization, HUVEC were allowed to bind and internalize FITC-coupled anti-P-selectin antibodies at 37 °C for 30 min. Internalization was stopped on ice and cells were then split. One aliquot was analysed directly and the second aliquot was treated additionally with anti-FITC antibodies for 30 min on ice to quench the remaining cell surface P-selectin signal. Internalization rates were calculated as percentages of mean fluorescence intensities (MFIs) obtained in the corresponding unquenched cells. Analysis used a FACSCalibur and CellQuest software (Becton Dickinson). Live cells were gated by using forward and side scatter characteristics, and only the fluorescence emissions of these cells were subsequently measured. Geometric MFIs were determined from 10,000 events. Non-specific binding was determined in cells treated with the appropriate isotype-matched antibodies and was subtracted from all values. For quantitative analysis of PSGL-1 cell surface expression, murine whole-blood samples were obtained by cardiac puncture and an anti-PSGL-1-PE antibody (2PH1, BD Biosciences) was added for 20 min at room temperature. After RBC lysis, the PSGL-1 surface expression on leukocytes was quantified by flow cytometry using FlowJo for data analysis (FacsCanto, BD Biosciences). Atomic force microscopy Topographical images of fixed HUVEC before and after incubation with anti-P-selectin antibodies were obtained using a Bioscope Catalyst AFM (Bruker Instruments, St. Barbara, CA, USA) and Nanoscope v.8.10 software. V-shaped OTR4 tips (Olympus) with a nominal spring constant of 0.02 N m −1 were used to image the surface of the cells. The force applied to the cantilever was adjusted manually to the lowest possible value necessary to maintain contact between the AFM tip and the sample (generally~50 pN). The feedback gains were optimized to obtain the best resolution in both topography and deflection images. Imaging was performed in fluid (PBS buffer) with 512 lines per screen. Line scan frequencies were 1–1.5 Hz. Data were processed and analysed with commercially available software (Scanning probe image processor, Image Metrology, Lyngby, Denmark). Super-resolution SIM Image stacks of single cells stained with anti-CD63 and anti-LAMP2 as well as appropriate fluorescently labelled secondary antibodies were recorded by conventional widefield fluorescence and super-resolution SIM [37] . Each stack consisted of nine individual images along the z axis. Quantitative image evaluation of individual cells was performed using the ImageJ software distribution FIJI ( http://fiji.sc/wiki/index.php/Fiji ). For each stack image, CD63 and LAMP2 signals were thresholded and quantified. In addition, LAMP2 signals over threshold were binarized and used as a mask to measure the CD63 signal intensity at the limiting membrane of endolysosomes. CD63 signal intensities originating from the CD63 fraction on membranes of intraluminal vesicles within the endolysosomes were determined by subtracting the signal at the limiting membranes from the overall CD63 intensities. Ratios of CD63 at the limiting membranes to CD63 on intralumenal membranes were calculated for 30 cells from three independent experiments. Quantification of VWF secretion HUVEC were grown to confluency on collagen-coated 24-well plates, serum starved overnight and then incubated for 20 min in fresh basal medium to measure the constitutive VWF secretion. Thereafter, WPB exocytosis was triggered by incubating the cells in histamine-containing basal medium for another 20 min. VWF secretion was then quantified as described [38] . Subcellular WPB fractionation HUVEC were scraped into ice-cold homogenization buffer (20 mM HEPES/KOH, pH 7.5, 5 mM EDTA and 250 mM sucrose) containing complete protease inhibitor cocktail (Roche, Basel, Switzerland), collected by centrifugation and lysed by passage through a 22-gauge needle. Postnuclear supernatants were then prepared by centrifugation at 1,000 g at 4 °C for 10 min, and volumes were adjusted to 3 ml with homogenization buffer. Postnuclear supernatants were loaded on discontinuous sucrose gradients (1.0 M: 2 ml, 1.1 M: 2 ml, 1.3 M: 2 ml, 1.6 M: 1.5 ml and 1.8 M: 1.5 ml) and centrifuged at 250,000 g for 90 min at 4 °C. The amounts of VWF and CD63 in each fraction were analysed by ELISA (CD63 determination used a kit from Hölzel Diagnostica, Cologne, Germany) and expressed as percentages of total VWF or CD63, respectively, calculated by summing up the VWF or CD63 amount of each fraction. ANXA8 targeting construct design The 3.1-kb left flanking region containing intron 1 genomic sequences, the 0.4-kb exon 2 genomic region together with intronic sequences and the 5.4-kb right flanking region containing exons 3–9 and genomic sequences were PCR amplified from mouse genomic DNA using oligonucleotides AN8_FLAdir3 (5′-TGTCGACGAGAAAAACCCTGTCCACGCTTAG-3′) and AN8_FLArev2 (5′-TGAATTCACACAGTTCTCATCCGCACCGT-3′); AN8_Exon2dir (5′-AGGATCCAACTGTGTGTGACCAGTCCGCTA-3′) and AN8_Exon2rev (5′-TAAGCTTATAACTTCGTATAGCATACATTATACGAAGTTATGAGGATGTGGGATGTGAGGC-3′, containing the exon 2 flanking LoxP site together with the HindIII site); and AN8_FLBdir2 (5′-TAAGCTTGGGCCCCCATTTTACTAAGTGACT-3′) and AN8_FLBrev (5′-TGCGGCCGCGGGGGATTGAATAGACAACATGAA-3′). All PCR products were subcloned, verified by sequencing and assembled into the final targeting construct (pAN8_targ. ; Fig. 7a-2 ). The pBluescript based plasmid backbone together with the negative selection marker (thymidine kinase cassette and diphtheria toxin gene) were added to the left flanking region. The positive selection marker (neomycin cassette flanked by two FRT sites and one LoxP site) was cloned as EcoRI–BamHI DNA fragment between left flanking region and exon 2. ES cell transfection and selection of targeted clones CV19 embryonic stem (ES) cells (passage 13 (129Sv × C57BL/6J)) were expanded in HEPES-buffered Dulbecco’s modified Eagle’s medium supplemented with 15% fetal bovine serum (PAA), nonessential amino acids, L -glutamine, β-mercaptoethanol, 1,000 U of recombinant leukaemia inhibitory factor (Merck Millipore) per ml, and antibiotics (penicillin (100 U ml) and streptomycin (100 μg ml −1 )). For electroporation, 2 × 10 7 cells were resuspended in 0.8 ml Capecchi buffer (20 mM HEPES; pH 7.4, 173 mM NaCl, 5 mM KCl, 0.7 mM Na 2 HPO 4 , 6 mM dextrose and 0.1 mM β-mercaptoethanol [39] . The targeting vector pAN8_targ. was linearized with NotI, and 55 μg of DNA was electroporated at 25 μF and 400 V in 0.8 mm electroporation cuvettes (Gene Pulser; Bio-Rad). After electroporation, cells were cultivated for 10 min at room temperature and plated onto 10 100-mm diameter culture dishes containing a gamma-irradiated monolayer of mouse primary G418-resistant fibroblast feeder cells. Thirty-two hours later, 350 μg of G418 (Invitrogen) per ml and 0.2 μM FIAU (1′-deoxy-2′-fluoro-β- D -arabinofuranosyl-5-iodouracil, Moravek Biochemicals and Radiochemicals, USA) were added. The medium was replaced every day, and colonies were picked and analysed 8 days after plating. DNA Southern blot analysis The HR probe (1,813 bp) was PCR amplified from mouse genomic DNA using oligonucleotides AN8_HRdir (5′-TGAGGACCCTATCCATGTGTGTA-3′) and AN8_HRrev (5′-CTTGGAAACTCTGAGGTAGCGTT-3′), subcloned and verified by sequencing. Approximately 5 μg of genomic ES cell clone DNA was digested with EcoRI, fractionated on 0.8% agarose gels and transferred to GeneScreen nylon membranes (NEN DuPont). The membranes were hybridized with a 32 P-labelled 1.8-kb probe containing sequences 5′ to the targeted homology (HR probe ( Fig. 7a-1 )) and washed with (final concentrations) 0.5 × SSPE (1 × SSPE is 0.18 M NaCl, 10 mM NaH 2 PO 4 and 1 mM EDTA, pH 7.7) and 0.5% sodium dodecyl sulphate at 65 °C. After a first screening, the correctly targeted event was verified by Southern blot analysis of DNA from positively targeted ES cells following digestion with HindIII (wt (+/+) allele 10,881 bp, targeted allele (fl) 7,198 bp). Blastocyst injection Correctly targeted ES cells from two independent clones (1H6 and 4F5) were injected into 3.5-day B6D2F1 blastocysts. Routinely, 12–14 ES cells were injected into one blastocoel. Blastocysts were kept in KSOM medium and then transferred into the uteri of 2.5-day pseudopregnant CD-1 foster mice. The mice carried pups to term. Chimeras were identified by their agouti coat colour contribution. For the germ-line transmission, high percentage male chimeras were cross-bred with female C57BL/6J mice. Tail biopsy DNA was digested with HindIII (wt allele 10,881 bp, targeted allele (fl) 7,198 bp, exon 2-deleted allele (Δ) 6,772 bp), and Southern blot analysis with the HR probe was used to detect the homologous recombinated ANXA8 locus. A homozygous floxed line was established and subsequently, anxA8 fl/fl mice were crossed with C57BL/6 pgk-Cre mice [40] . Homozygous anxA8 KO mice were obtained by further crossing with anxA8 fl/fl mice. All mouse procedures were performed in compliance with the guidelines for the welfare of experimental animals issued by the Federal Government of Germany. Animals were kept in specific pathogen-free animal facilities and housed in standard individually ventilated cages (IVC). Pups were weaned at 19–23 days after birth, and females were kept separately from males. General health checks were performed regularly in order to ensure that any findings were not the result of deteriorating physical conditions of the animals. Detection of ANXA8-deleted allele by PCR and western blotting The genotype of each mouse was determined by PCR on tail genomic DNA. A primer pair (5′-GAGTTTATTTCCACCCATCCTGCTGTA-3′ and 5′-AGAGCCAGTGTGATGCTGTAAGTAAC-3′) was designed that yields 510 bp, 2.4 kb and 2 kb PCR fragments of the wt (+), the LoxP flanked (fl) and the exon 2 deleted (Δ) alleles, respectively. Tail tips were incubated overnight at 56 °C in lysis buffer (100 mM Tris–HCl, pH 8.5, 5 mM EDTA, 200 mM NaCl and 0.2% SDS) containing proteinase K. After RNAse digestion and extraction with phenol/chloroform/isoamyl alcohol, genomic DNA was dissolved in 200 μl buffer (10 mM Tris–HCl, pH 8.5). Each of the genomic DNA preparations was submitted to PCR amplification and analysed on a 1.5% agarose gel. For western blotting analysis, tail tissue frozen in liquid nitrogen was homogenized in tissue extraction buffer (20 mM Tris–HCl, pH 7.4, 1% NP-40, 10% glycerol, 137 mM NaCl, 10 mM EDTA and 1 mM EGTA) containing protease inhibitors. Protein concentration in the extracts was determined by the Bradford method, and 1 μg samples were subjected to 12% SDS PAGE. AnxA8 protein levels were visualized by probing the blots with polyclonal rabbit antibodies raised against murine anxA8 (a kind gift from Torsten Stein, University of Glasgow, UK). The blot was stripped and reprobed with the HH7 anti-anxA2 antibody. α-Tubulin was used as a loading control. Intravital microscopy Intravital microscopy was performed as described previously [41] . Briefly, male mice 8–14 weeks of age were anaesthetized with ketamine (125 mg kg −1 ) and xylazine (12.5 mg kg −1 ). To induce inflammation, the cremaster muscle was exteriorized and superperfused with 5 nM KC (CXCL1; R&D Systems, Wiesbaden-Nordenstadt, Germany) for 1 h. Intravital microscopy was carried out on an upright microscope (Axioskop; Carl Zeiss, Goettingen, Germany) with a × 40 saline immersion objective, NA 0.75. Movies were obtained using a digital camera (AxioCam MRm, Carl Zeiss) and recorded and analysed using digital video software (ZEN 2012; Carl Zeiss). Leukocyte rolling flux and the number of adherent leukocytes were determined by transillumination intravital microscopy. Rolling velocity was calculated by measuring the distance covered by rolling cells with ImageJ (NIH), divided by the time of rolling, and is given as μm s −1 . All animal experiments were approved by the Landesamt für Natur, Umwelt und Verbraucherschutz Nordrhein-Westfalen and were carried out according to the German legislation on protection of animals. Statistical analysis Sample size required to detect moderate-to-strong effects was estimated by power analysis using G*Power 3.1 (ref. 42 ). Statistical significance of the results was evaluated by unpaired Student’s t -test or one-way analysis of variance (ANOVA) followed by Tukey’s or Bonferroni’s multiple comparison test using GraphPad Prism version 4.00 (GraphPad software, San Diego, CA, USA). How to cite this article: Poeter, M. et al . Annexin A8 controls leukocyte recruitment to activated endothelial cells via cell surface delivery of CD63. Nat. Commun. 5:3738 doi: 10.1038/ncomms4738 (2014).